Stable, active CO2reduction to formate via redox-modulated stabilization of active sites Electrochemical reduction of CO 2 (CO 2 R) to formic acid upgrades waste CO 2 ; however, up to now, chemical and structural changes to the electrocatalyst have often led to the deterioration of performance over time. Here, we find that alloying p-block elements with differing electronegativities modulates the redox potential of active sites and stabilizes them throughout extended CO 2 R operation. Active Sn-Bi/SnO 2 surfaces formed in situ on homogeneously alloyed Bi 0.1 Sn crystals stabilize the CO 2 R-to-formate pathway over 2400 h (100 days) of continuous operation at a current density of 100 mA cm −2 . This performance is accompanied by a Faradaic efficiency of 95% and an overpotential of ~ −0.65 V. Operating experimental studies as well as computational investigations show that the stabilized active sites offer near-optimal binding energy to the key formate intermediate *OCHO. Using a cation-exchange membrane electrode assembly device, we demonstrate the stable production of concentrated HCOO – solution (3.4 molar, 15 wt%) over 100 h. Electrochemical CO 2 reduction (CO 2 R) driven by electrical energy converts CO 2 into low carbon footprint chemicals and fuels [1] . Among CO 2 R products, formic acid (HCOOH) or formate (HCOO – ) is used in pharmaceutical, electrolytic metallurgy, leather, and fuel cell applications [2] , [3] , [4] , [5] , [6] . HCOO – has a high market value per energy (cents/kWh) [7] , making it a candidate of particular interest. Conventionally, HCOO – is produced from the hydrolysis of methyl formate, which uses CH 3 OH and CO as starting materials. This chemical reforming process requires strict reaction conditions and high energy input [8] , [9] , [10] . In contrast, CO 2 R requires only CO 2 , water, and electrical energy [7] , [11] , [12] . Unfortunately, to date, CO 2 R catalysts and systems favouring HCOO – have not achieved the required combination of high selectivity (Faradaic efficiency (FE)) [13] , high reaction rate (current density) [13] , high energy efficiency (EE) [14] , and, in particular, long-term stability. Among electrocatalytic materials studied, Sn is a promising candidate owing to its low cost and planetary abundance [15] , [16] . Sn has strong binding energy for *OCHO, and this favours the first-step CO 2 hydrogenation in CO 2 -to-formate conversion [17] , [18] . The second step electron transfer requires high energy to reduce *OCHO to HCOO – , resulting in a large overpotential and consequently a low EE. Sn has medium binding energy to *COOH and *H, which makes it difficult to fully suppress CO and H 2 generation; the FE for HCOO – has therefore been limited to 80–85%. Recent studies of Sn-based core-shell structures, including Ag-Sn [19] , Cu-Sn [20] , Bi-Sn [21] , and phase-segregated bimetallic systems [22] , [23] , showed improved FE for HCOO – . Further improvement of the HCOO – production rate and cathodic energy efficiency (CEE) relative to current benchmarks (Supplementary Table 4 ) requires precise control of the elemental distributions in the active sites. In particular, knowledge of the electrochemical stability of Sn and Sn-based materials in aqueous electrolytes at different pH is lacking; indeed, among reported formate catalysts, it has been challenging to combine optimal adsorption energetics for intermediate binding with sites stable against reconstruction [13] , [14] , [15] , [16] . Here, we present active Sn-Bi/SnO 2 surfaces that are grown conformally on uniformly alloyed Bi 0.1 Sn crystals. 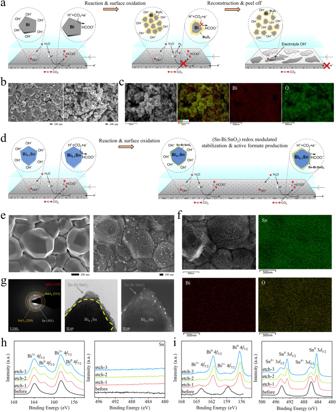Fig. 4: Structural and elemental analyses of the Bi and Bi0.1Sn electrocatalyst before and after CO2 reduction at pH 11 and a current density of 100 mA cm-2. aSchematic of Bi reconstruction during the electrochemical reaction.bSEM results of the as-prepared Bi nanoplates, and the reconstructed Bi/Bi2O3core/shell nanoparticles after 70 h of reaction.cSEM-EDX elemental mapping results of the Bi/Bi2O3catalysts after 70 h of reaction.dSchematic of a redox-modulated Bi0.1Sn/SnO2surface on Bi0.1Sn during the electrochemical reaction.eSEM results of the as-prepared Bi0.1Sn crystals, and the (Bi0.1Sn/SnO2)/Bi0.1Sn particles over 100 h of reaction.fSEM-EDX elemental mapping results of the (Sn-Bi/SnO2)/Bi0.1Sn catalyst over 100 h of reaction.gThe SAED pattern, bright-field and dark-field TEM images of the Sn-Bi/SnO2catalysts over 100 h of reaction.hXPS depth profiles of the post-reaction Bi after 50-h CO2reduction at 100 mA cm−2in 1 M KHCO3and KOH electrolytes at pH = 11.iXPS depth profile of the post-reaction Bi0.1Sn after 100-h CO2reduction at 100 mA cm−2in 1 M KHCO3and KOH electrolytes at pH = 11. The black, red, green and blue lines represent the XPS data before etching (black) and after different time courses of soft Ar etching (red, green, blue), respectively. The etched depth in each soft Ar etching is ~3–5 nm. These surfaces support the stable reduction of CO 2 to formate over a period in excess of 2400 h (100 days) of continuous operation, with a near-unity formate FE of over 95% and a CEE exceeding 70% at a current density of 100 mA cm −2 in 1 M potassium bicarbonate (KHCO 3 ) and potassium hydroxide (KOH) electrolytes at pH 11. This stability and CEE is significantly improved compared to literature benchmarks [13] , [24] , [25] , [26] , [27] . The selectivity and energy efficiency obtained to meet the performance required for a positive net present value in an economic analysis of formate production [11] . Computational studies reveal that, across a wide range (1.5–12.5%) of Bi incorporation into Sn, the facets of Sn-Bi alloys and Sn-Bi/SnO 2 composites provide sites with near-optimal binding energy to *OCHO. This approach lowers the reaction energy in CO 2 -to-formate conversion. The by-products CO and H 2 are suppressed due to their increased reaction energy on Sn-Bi alloys. The redox-modulated Sn-Bi/SnO 2 surfaces remain active and protect Bi 0.1 Sn catalysts against corrosion or reconstruction during extended CO 2 R. We further demonstrate stable production of 3.4 molar (15 wt%) HCOO – (formate) solution of over 100 h at a constant current density of 60 mA cm −2 with an average full-cell EE of ~27% in a membrane electrode assembly (MEA) system based on a cation-exchange membrane (CEM), highlighting that Bi 0.1 Sn catalysts are reliable for long-lasting HCOO – (formate) production in different CO 2 R systems. Characterization We used thermal evaporation to produce Bi x Sn ( x = 0.1, 0.2, 0.3), Bi, and Sn precatalysts on polytetrafluoroethylene (PTFE) gas diffusion substrates (Supplementary Fig. 1 ). Dense and compact particle-film layers were formed for all Bi x Sn ( x = 0.1, 0.2, 0.3), Bi, and Sn catalysts, ensuring electrical conductivity for CO 2 R (Supplementary Fig. 2 ). The particle size is 200–300 nm for the Bi and 1–1.5 μm for the Sn catalyst. Bi 0.2 Sn and Bi 0.3 Sn possess similar particle sizes of 1–1.5 μm to that of Sn, but they fail to form a uniform alloy; Bi precipitates over a large area (Supplementary Figs. 3 , 4 ). Bi 0.1 Sn forms uniform crystals with particle sizes of 700–1000 nm, as confirmed by scanning electron microscopy (SEM), transmission electron microscopy (TEM) images, and scanning transmission electron microscopy–energy dispersive spectroscopy (STEM-EDS) elemental mapping in Fig. 1b, c, e . The selected area electron diffraction (SAED) pattern of Bi 0.1 Sn exhibits distinct single-crystal diffraction spots corresponding to the Sn plane indexes (Fig. 1d ), suggesting that Bi is incorporated into the Sn crystals. The facets exposed are primarily (200) and (101), consistent with the observations from high-resolution TEM analysis (Fig. 1c ). 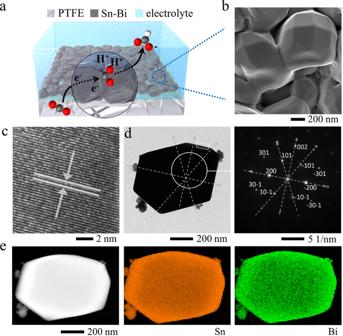We carried out STEM-EDS, SEM-EDS, and XPS analyses, and obtained similar Bi concentrations of ~10 at.% for the Bi 0.1 Sn catalyst (Supplementary Figs. Fig. 1: Structural and elemental analyses of Bi0.1Sn electrocatalysts. aSchematic of Bi0.1Sn electrocatalyst on a polytetrafluoroethylene gas diffusion layer for electroreduction of CO2.bSEM,cHRTEM,dTEM, SAED, and,eSTEM, EDS analyses of Bi0.1Sn electrocatalyst. The high-resolution TEM image in (c) shows the lattice fringes corresponding to the Sn (200) facet. The dashed box in (d) is the location to take the HRTEM. 5 – 9 and Table 1 ), suggesting that Bi and Sn are uniformly distributed from the surface to the bulk. Fig. 1: Structural and elemental analyses of Bi0.1Sn electrocatalysts. a Schematic of Bi 0.1 Sn electrocatalyst on a polytetrafluoroethylene gas diffusion layer for electroreduction of CO 2 . b SEM, c HRTEM, d TEM, SAED, and, e STEM, EDS analyses of Bi 0.1 Sn electrocatalyst. The high-resolution TEM image in ( c ) shows the lattice fringes corresponding to the Sn (200) facet. The dashed box in ( d ) is the location to take the HRTEM. Full size image Table 1 The molar concentration of Bi and Sn in the Bi 0.1 Sn obtained by XPS, SEM-EDS, and TEM-EDS analyses. Full size table Density functional theory (DFT) calculations In light of the above characterizations, we built models and performed DFT studies to calculate the reaction energy on Bi, Sn, and Bi y Sn 64 ( y = 1, 2, 4, 8) surfaces (details in Supplementary Figs. 10 – 15 and Supplementary Table 1 ). As shown in Fig. 2a , the production of CO, CH 4 , and other C 2+ hydrocarbons generally proceeds via the *COOH intermediate pathway [28] , [29] . *COOH adsorption requires the outer shell electrons of catalysts to have both energy that matches the LUMO energy of CO 2 , and electronic orbitals that overlap with molecular orbitals of the C–O π bond. Production of HCOO – often occurs via the *OCHO intermediate pathway [14] , [18] . This requires catalysts to possess suitable binding energy to O. Bi and Sn are both p-block metals that, as shown in Fig. 2b, d , display significantly uphill reaction energy to *COOH compared to that to *OCHO, indicating that HCOO – is the major product. Fig. 2: DFT calculations. a Possible pathways of electrochemical CO 2 reduction. The top panel shows the *COOH pathway to produce CO, CH 4 , or C 2+ hydrocarbons. The bottom panel shows the *OCHO pathway to produce HCOO – . Bi, Sn, C, O, and H atoms are represented by green, yellow, grey, red, and white spheres, respectively. b Reaction energy for CO formation on Bi (003), Sn (200), and Bi 4 Sn 64 (200) surfaces without applying any external potential ( U = 0 eV). c The volcano plot describing *OCHO adsorption energy versus CO 2 -to-HCOO – reaction energy. d Reaction energy for HCOO – formation on Bi (003), Sn (200), and Bi y Sn 64 ( y = 1, 2, 4, 8) surfaces without applying any external potential ( U = 0 eV). 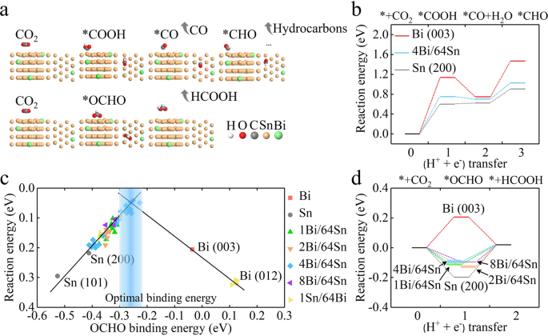Full size image Since the intermediate *OCHO is energetically more favourable than *COOH on Bi, Sn, and Bi 0.1 Sn surfaces, we examined their reaction energy for HCOO – production in detail. Fig. 2: DFT calculations. aPossible pathways of electrochemical CO2reduction. The top panel shows the *COOH pathway to produce CO, CH4, or C2+hydrocarbons. The bottom panel shows the *OCHO pathway to produce HCOO–. Bi, Sn, C, O, and H atoms are represented by green, yellow, grey, red, and white spheres, respectively.bReaction energy for CO formation on Bi (003), Sn (200), and Bi4Sn64(200) surfaces without applying any external potential (U= 0 eV).cThe volcano plot describing *OCHO adsorption energy versus CO2-to-HCOO–reaction energy.dReaction energy for HCOO–formation on Bi (003), Sn (200), and BiySn64(y= 1, 2, 4, 8) surfaces without applying any external potential (U= 0 eV). Figure 2d reveals that Bi (003) tends to bind *OCHO too weakly, that Sn (002) may bind *OCHO too strongly, and that of the calculated BiSn slabs, Bi 4 Sn 64 and Bi 8 Sn 64 show the optimal binding energy to *OCHO of near to –0.13 eV, indicating low reaction energy for the CO 2 -to-HCOO – conversion. We plotted the reaction energy of different catalyst archetypes as a function of their adsorption energy to *OCHO at 298 K and 1 atm. (Fig. 2c ). We took an average of the binding energy on enumerated possible configurations and present the averaged binding energy in Fig. 2d . Bi y Sn 64 ( y = 1, 2, 4, 8), with a relatively wide range of Bi ratios in different Sn facets, exhibits an abundance of adsorption sites with improved *OCHO binding energy that enhances CO 2 reduction (DFT calculation details are given in Supplementary Figs. 12 – 15 ). The volcano relationship predicts that Bi 4 Sn 64 (incorporation of 6.25% Bi into Sn) may be the most active (Supplementary Table 2 ). We further find that Bi 4 Sn 64 elevates the reaction energy to CO and H 2 , suppressing the generation of CO, H 2 , and C 2+ hydrocarbons (Fig. 2b and Supplementary Fig. 11 ). In summary, our computational simulations point to the alloying of Sn with Bi as a strategy to enhance HCOO – production. CO 2 R in aqueous flow cells The CO 2 R performance of Bi x Sn alloys ( x = 0.1, 0.2, 0.3), as well as pure Bi or Sn control samples, was first evaluated in 1 M KOH electrolyte (pH = 14) in a flow-cell electrolyser. Ag/AgCl electrodes were used as the reference electrodes, and commercial Ni foams were used as the anodes for the water oxidation reaction in a three-electrode setup. Linear sweep voltammetry (LSV) curves obtained from 0 V to –2 V vs. reversible hydrogen electrode (V RHE ) show that Bi 0.1 Sn has the most positive onset potential for CO 2 R (Fig. 3a and Supplementary Fig. 16a ). This is consistent with the DFT calculations that incorporating 1.5–12.5% Bi into Sn lowers the reaction energy in the electrochemical CO 2 -to-formate conversion (Fig. 2 ). A rapid increase of the cathodic current is observed with Bi 0.1 Sn at potentials more negative than –0.5 V RHE . To study the electrochemical characteristics of the Bi 0.1 Sn, Bi, and Sn catalysts, we carried out the electrochemical active surface area (ECSA), and electrochemical impedance spectroscopy (EIS) analyses [30] . The estimated ECSAs of Bi and Bi 0.1 Sn are twice as large as that of Sn (Supplementary Fig. 17 ). Also, Bi 0.1 Sn has the lowest interface resistance (Supplementary Fig. 18 ). These results confirm that Bi 0.1 Sn reduces the potential loss and, consequently, improves the CEE. Fig. 3: CO2 electroreduction performance using Bi0.1Sn, Bi, and Sn catalysts. a Linear sweep voltammetry curves of Bi 0.1 Sn, Bi, and Sn in 1 M KOH electrolyte. b The corresponding formate FEs under different current densities. c Linear sweep voltammetry curves. d The corresponding formate FEs in 1 M KHCO 3 and KOH electrolytes at different pH (pH = 8, 10, 11, 12, 13, and 14) at a current density of 100 mA cm −2 . e The CO 2 -reduction chronopotentiometry curve (blue line), CO 2 -to-formate FE (blue dots), and CO 2 -to-formate half-cell energy conversion efficiency (purple dots) in 1 M KHCO 3 and KOH electrolyte at pH = 11 at an applied current density of 100 mA cm −2 . f Comparison of our work with previously published data. Error bars correspond to the standard deviation of five independent measurements. Full size image To quantify the FEs of CO 2 R products, Bi x Sn ( x = 0.1, 0.2, 0.3), Bi, and Sn catalysts were evaluated in a chronopotentiometry mode by applying current densities of 100, 200, and 300 mA cm −2 . Gaseous and liquid products were quantified by gas chromatography (GC) and nuclear magnetic resonance (NMR), respectively. As shown in Fig. 3b and Supplementary Fig. 16b , the Bi 0.1 Sn catalyst shows over 95% FE for HCOO – in a wide range of current densities. Only a small amount of H 2 and CO was detected, and no other liquid products were formed (Supplementary Figs. 19 , 20 ). A CO 2 -to-formate CEE of ~75% was achieved at pH 14 at 100 mA cm −2 . 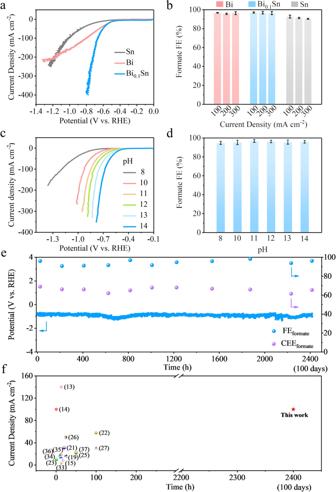Under similar conditions, Bi 0.2 Sn, Bi 0.3 Sn, and Bi catalysts produce 95% FE for HCOO – , but they require a more negative potential for the same current density (Supplementary Fig. Fig. 3: CO2 electroreduction performance using Bi0.1Sn, Bi, and Sn catalysts. aLinear sweep voltammetry curves of Bi0.1Sn, Bi, and Sn in 1 M KOH electrolyte.bThe corresponding formate FEs under different current densities.cLinear sweep voltammetry curves.dThe corresponding formate FEs in 1 M KHCO3and KOH electrolytes at different pH (pH = 8, 10, 11, 12, 13, and 14) at a current density of 100 mA cm−2.eThe CO2-reduction chronopotentiometry curve (blue line), CO2-to-formate FE (blue dots), and CO2-to-formate half-cell energy conversion efficiency (purple dots) in 1 M KHCO3and KOH electrolyte at pH = 11 at an applied current density of 100 mA cm−2.fComparison of our work with previously published data. Error bars correspond to the standard deviation of five independent measurements. 16 b, 21 and Supplementary Table 3 ). The Sn catalyst produces an FE of ~85% for HCOO – , along with a constant total FE of ~15% for H 2 and CO. It also requires a more negative potential to reach 100 mA cm −2 , and thus the CEE for HCOO – is limited to 50%. To assess the stability of the Bi 0.1 Sn catalyst during CO 2 R, carbon nanoparticles (NPs) and graphite were coated on the Bi 0.1 Sn/PTFE electrode to form a hybrid structure of graphite/carbon NPs/Bi 0.1 Sn/PTFE. This structure enables uniform distribution of the electrolyte and electrical current over the Bi 0.1 Sn surfaces [31] , [32] . Note that the coated carbon nanoparticles and graphite are not CO 2 R electrocatalysts and they don’t produce any formate under our CO 2 R operating conditions. Importantly, we coated carbon nanoparticles and graphite for all the Bi, Sn, and Bi 0.1 Sn catalysts, comparing their CO 2 R activity under the same working conditions. We are therefore certain that the performance obtained solely represents the properties of each catalyst. We also kept the electrolyte pH unchanged during the long-term CO 2 R stability test so that the CO 2 R results are all compared under the same pH conditions. In our studies, Bi 0.1 Sn catalyst produces HCOO – with an FE exceeding 95% for over 170 h at 100 mA cm −2 and an overpotential of ~–0.5 V RHE in 1 M KOH electrolyte (Supplementary Fig. 22 ). Control experiments for Bi and Sn samples using similar carbon/graphite coatings led to both lower CEEs and worse stability within 50–70 h (see Supplementary Methods and Supplementary Figs. 23 – 25 ). To evaluate the effect of pH on the activity and stability of CO 2 R, we studied the performance of Bi 0.1 Sn catalysts in KHCO 3 and KOH electrolytes at different pH levels (see the Supplementary Methods for details). As shown in Supplementary Fig. 26 , the formate FEs are above 90% at all pH (8–14) at current densities from 25 to 300 mA cm −2 . This indicates that the formate FE is directly related to the properties of catalysts because the CO 2 R kinetics are more favourable than those of the competing hydrogen evolution reaction under these working conditions. The use of alkaline electrolytes also shifts the working potential positively with the increase of electrolyte pH. As shown in Figs. 3 c, 3d and Supplementary Fig. 27, the CEEs for HCOO – are above 70% at 100 mA cm −2 at pH greater than 11. We performed 100-hour stability tests at varying pH (11–14) at a current density of 100 mA cm −2 and analysed their surface morphology, composition, and other material properties after the reaction by SEM, XRD, XPS, and EDX (Supplementary Figs. 28 – 31 ). At pH 11, the morphology change is minor compared to those at higher pH levels after 100 h of operation. This is in line with the Pourbaix diagram (Supplementary Fig. 32 ), in which both metallic Bi and Sn are cathodically protected at potentials more negative than –0.35 V RHE at pH 11. The self-corrosion potentials of Bi 0.1 Sn catalysts at pH 11–14 in Supplementary Fig. 34 indicate that, thermodynamically, the tendency of corrosion increases with the increase of pH. Remarkably, we achieved efficient CO 2 R over 2400 h (100 days) at pH 11 with stable 70% CEE (Fig. 3e ). A full-cell EE of 35% (without IR correction) was obtained using unmodified, commercial Ni foams as anodes for the water oxidation reaction in a flow-cell system (Supplementary Fig. 35 ). This is significant in developing CO 2 R electrolysers that meet the long operational stability requirements for commercialization [12] of at least 1000 h with current densities exceeding 100 mA cm −2 . Ours is the first demonstration of CO 2 R stability achieving this goal. To put our results in a broader context, we plotted our data with reported values [13] , [14] , [15] , [19] , [21] , [22] , [23] , [25] , [26] , [27] , [33] , [34] , [35] , [36] , [37] in Fig. 3f . The stability and CEE at current densities ≥ 100 mA cm −2 we achieved outperform literature benchmarks by two orders of magnitude, indicating a critical milestone in the field of CO 2 R field. We compared the CO 2 R performance of Bi and Sn at 100 mA cm −2 and in 1 M KHCO 3 and KOH electrolytes at pH 11. Sn produces ~80% FE for HCOO – with a constant total FE of ~20% for H 2 and CO. The hydrogen evolution reaction increases and HCOO – decreases throughout electrolysis (Supplementary Fig. 37 ). Bi produces 95% FE for HCOO – , but the CEE is much lower (Supplementary Figs. 36 , 37 ). We found that the stability of Bi was poor: We performed 10 independent tests for Bi samples in an aqueous system with a continuous operation of 100 h. We observed performance decay and peeling off of Bi in all tests (Supplementary Fig. 38 ). To diagnose the origins of catalyst instability during CO 2 R, we compared Bi and Bi 0.1 Sn catalysts before and after the reactions. After the 70-h test, the original 200–500 nm Bi crystals were completely reconstructed to 20–50 nm nanoparticles with a large amount of O on the surfaces (Fig. 4a–c ). SEM-EDX and HRTEM analyses reveal that polycrystalline Bi 2 O 3 was formed on Bi, which is in line with the XRD results for Bi after the reaction; the yellow line in the HRTEM image indicates the boundary between the Bi bulk and the Bi 2 O 3 surface (Fig. 4b, c and Supplementary Figs. 39 – 40 ). This chemical and structural transformation is associated with effects involving (i) the non-uniform distribution of electrical potential on the surfaces during the reaction [38] , [39] and (ii) the existence of OH – near Bi at pH 11 to make redox reactions between Bi and Bi 2 O 3 continuously occur. Metastable Bi failed to form equilibrated phases on the surfaces and, thus, Bi was continuously reconstructed during the reaction. The reconstructed Bi 2 O 3 /Bi nanoparticles show increased electrical resistance to decrease the overall performance. As shown in the XPS depth profile studies, Bi 3+ was detected on the 50h-reaction Bi throughout three rounds of the 3–5 nm soft Ar etching (Fig. 4h ). This gives evidence that Bi 3+ is presented in the bulk of the 50h-reaction Bi sample. In contrast, when we studied the evaporated Bi catalyst before reaction, Bi 3+ disappeared after one round of ~3–5 nm soft Ar etching, indicating that the top surface Bi was oxidized in air and no bulk oxidation was observed (Supplementary Fig. 41 ). DFT studies in Supplementary Fig. 42 reveal that the Bi 2 O 3 (002) and (210) facets largely shift the *OCHO reaction energy to ~–0.83 and ~0.30 eV, which is either too strong or too weak for the reaction as predicted by the volcano relationship in Fig. 2c . Taking these together with SEM, TEM, and electrochemical analyses for the Bi control samples before and after the reaction in Fig. 4b, c and Supplementary Figs. 38 , 39 , we conclude that Bi reconstructed to Bi 2 O 3 /Bi during the reduction, which leads to performance degradation and eventually catalyst peeling off. Fig. 4: Structural and elemental analyses of the Bi and Bi0.1Sn electrocatalyst before and after CO2 reduction at pH 11 and a current density of 100 mA cm -2 . a Schematic of Bi reconstruction during the electrochemical reaction. b SEM results of the as-prepared Bi nanoplates, and the reconstructed Bi/Bi 2 O 3 core/shell nanoparticles after 70 h of reaction. c SEM-EDX elemental mapping results of the Bi/Bi 2 O 3 catalysts after 70 h of reaction. d Schematic of a redox-modulated Bi 0.1 Sn/SnO 2 surface on Bi 0.1 Sn during the electrochemical reaction. e SEM results of the as-prepared Bi 0.1 Sn crystals, and the (Bi 0.1 Sn/SnO 2 )/Bi 0.1 Sn particles over 100 h of reaction. f SEM-EDX elemental mapping results of the (Sn-Bi/SnO 2 )/Bi 0.1 Sn catalyst over 100 h of reaction. g The SAED pattern, bright-field and dark-field TEM images of the Sn-Bi/SnO 2 catalysts over 100 h of reaction. h XPS depth profiles of the post-reaction Bi after 50-h CO 2 reduction at 100 mA cm −2 in 1 M KHCO 3 and KOH electrolytes at pH = 11. i XPS depth profile of the post-reaction Bi 0.1 Sn after 100-h CO 2 reduction at 100 mA cm −2 in 1 M KHCO 3 and KOH electrolytes at pH = 11. The black, red, green and blue lines represent the XPS data before etching (black) and after different time courses of soft Ar etching (red, green, blue), respectively. The etched depth in each soft Ar etching is ~3–5 nm. Full size image In contrast, the Bi 0.1 Sn catalyst remains stable during the long CO 2 R operation under the same working conditions. After our tests, Bi 0.1 Sn remains intact on PTFE with morphology preserved (Fig. 4d–f and Supplementary Fig. 43 ). Dark-field and bright-field TEM images with SAED patterns and HRTEM visualized conformal ~20–50 nm SnO 2 /Sn-Bi mixture layers on Bi 0.1 Sn surfaces (Fig. 4g and Supplementary Figs. 44 – 46 ). The SAED patterns show a polycrystalline nature of surface SnO 2 , in line with the XRD results (Supplementary Figs. 47 , 44c ). We carried out calculations of different initial configurations with O involved in the Sn-Bi system on the surface (Supplementary Fig. 48 ). The results reveal that the homogeneously alloyed Bi 0.1 Sn crystal with few O atoms involved on the surfaces shows similar catalytic performance to that of the metallic Bi 0.1 Sn crystal. DFT studies also reveal that the SnO 2 (110) facet remains active for HCOO – production with the optimal binding energy of ~–0.15 eV for *OCHO (Supplementary Fig. 42 ). As shown in the XPS depth profiles (Fig. 4i and Supplementary Fig. 49 ), after a round of ~ 3–5 nm soft Ar etching, Bi 0 , Sn 0 and Sn 4+ were observed in the consequent three rounds of the 3–5 nm soft Ar etching. The electrochemical redox potentials of Bi/Bi 3+ and Sn/Sn 4+ are 
    Bi_2O_3+3H_2O+6e ⇌  2Bi+6OH^- -0.46 V
 (1) 
    SnO_2+2H_2O+4e ⇌ Sn+4OH^- -0.945 V
 (2) This suggests that Sn should be oxidized before Bi. A redox-modulated balance between Sn and SnO 2 was formed on the bimetallic active sites on the surface during CO 2 R. The redox modulation between Sn/Sn 4+ protects the active BiSn:SnO 2 against corrosion. We, therefore, suggest that we in situ formed immobilized, conformal and active BiSn:SnO 2 surfaces during CO 2 reduction, being stable against chemical and structural change throughout extended CO 2 R reaction over 2400 h of continuous operation. After 2400 h, we observed densely packed Bi 0.1 Sn particles over the electrode with clear surface Bi and Sn signals identified by XPS (Supplementary Fig. 50 ). No significant leaching of Bi and Sn into solution was detected via inductively coupled plasma atomic emission spectroscopy (ICP-AES) analysis (Supplementary Fig. 51 ). We also provide SEM images and performance curves of Bi 0.1 Sn and Bi after different times taken from the stability tests as shown in Supplementary Fig. 52 . We witness no peeling of the catalyst during the 2400 h test. Note that a stable and efficient CO 2 R device requires stable and efficient reactions of CO 2 R and water oxidation. On the cathode side, Bi 0.1 Sn catalysts deliver excellent CO 2 R stability and activity via redox-modulated stabilization of active sites. On the anode side, it is vital to improving the stability and efficiency of the catalysts. CO 2 R in MEA systems To produce concentrated HCOO – solutions, we assessed the CO 2 R performance of Bi, Sn, and Bi 0.1 Sn catalysts in an MEA system (Fig. 5a, b ). We first used an anion-exchange membrane (AEM) to test the MEA performance. As shown in Fig. 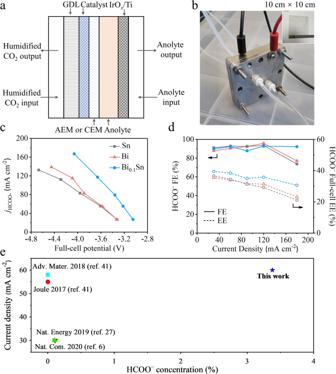Fig. 5: CO2electroreduction performance in anion-exchange membrane (AEM)-based MEA systems. aSchematic of the MEA configuration.bThe optical image of an MEA device.cCurrent densities vs. applied potentials of Bi, Sn, and Bi0.1Sn in AEM-based MEA systems.dHCOO–FEs and EEs of Bi, Sn, and Bi0.1Sn at different current densities in AEM-based MEA systems.eComparison of our data with literature benchmarks (We plot the concentration values obtained in the longest duration tests in each report). 5c, d , and Supplementary Table 5 , Bi 0.1 Sn produced over 90% FE for HCOO – in a wide range of current densities from 30 to 180 mA cm −2 . A peak FE for HCOO – of 97.8% was achieved at a current density of 120 mA cm −2 with a full-cell potential (without IR correction) of –3.6 V and a full-cell EE of 36%. As control experiments, pristine Bi and Sn delivered peak HCOO – FEs of 95.8% and 93.5% at the same current density of 120 mA cm −2 , but they required more negative potentials of –4.1 V and –4.3 V. As a result, the full-cell EEs for the MEAs using Bi and Sn catalysts were both lower, 31% and 29%, respectively. LSV curves confirmed the CO 2 R performance of Bi 0.1 Sn surpassed those of Bi and Sn in AEM-based MEA (Supplementary Fig. 53 ). Fig. 5: CO 2 electroreduction performance in anion-exchange membrane (AEM)-based MEA systems. a Schematic of the MEA configuration. b The optical image of an MEA device. c Current densities vs. applied potentials of Bi, Sn, and Bi 0.1 Sn in AEM-based MEA systems. d HCOO – FEs and EEs of Bi, Sn, and Bi 0.1 Sn at different current densities in AEM-based MEA systems. e Comparison of our data with literature benchmarks (We plot the concentration values obtained in the longest duration tests in each report). Full size image We then sought to translate the champion performance of Bi 0.1 Sn to a CEM-based MEA electrolyser as a strategy to minimize the crossover of HCOO – (formate) to the anode side to producing a concentrated HCOO – solution at the cathodic stream (HCOO – : 3.4 molar, 15 wt%). Replacing AEM with CEM likely changed the local pH near the catalyst surfaces during the reaction, leading to a shift of peak HCOO – FE to relatively lower current densities [7] , [40] . By using a high anolyte flow rate of 15 mL/min., we obtained a peak HCOO – FE of ~90% at 60 mA cm −2 with Bi 0.1 Sn (Supplementary Fig. 54 and Supplementary Table 5 ). We then optimized the single-pass flow rate of anolyte (0.1 M KHCO 3 ) to 1.5 mL/min. to promote the HCOO – concentration at the cathodic liquid stream. This optimization established a balance between membrane hydration and K + availability near the catalyst surface, enabling the collection of concentrated HCOO – directly from the cathodic stream. We obtained an average HCOO – FE of 82% (or 4.49 mmol/h) at 60 mA cm −2 during 100 h of CO 2 R with an average HCOO – concentration of 3.4 molar (15 wt%) (Supplementary Fig. 55 ). This represents a 30-fold improvement in HCOO – concentration with 100-hour stability along with a 2-fold increase in current density compared to the literature benchmarks reported in duration tests [6] , [27] , [41] , [42] (Fig. 5e ). We present redox-modulated, stable, and active Sn-Bi/SnO 2 surfaces on uniformly alloyed Bi 0.1 Sn crystals, and these catalysts show a combination of high activity and performance stability in the CO 2 -to-HCOO – reduction exceeding 2400 h (100 days) of continuous operation. We use DFT calculations to explain that the stabilized active sites improve *OCHO binding energy and fine-tune *COOH and *H binding energy for selective HCOO – production. We show stable production of concentrated HCOO – (formate) of 3.4 molar with Bi 0.1 Sn catalysts in a solid-state CEM-based MEA system over 100 h. Our demonstration of a stable catalyst and system is a crucial step to deliver reliable and long-lasting CO 2 R technology. Further efforts will be necessary to increase CO 2 single-pass yield and to the broader applicability of this system in the production of other C 2 + liquid fuels and beyond. Synthesis Bi x Sn ( x = 0.1, 0.2, 0.3), Bi, and Sn electrocatalysts were synthesized using thermal evaporation (SKY-RH400). In brief, to fabricate the Bi x Sn ( x = 0.1, 0.2, 0.3) catalysts, different amounts of Sn and Bi were co-evaporated onto the PTFE substrates under the pressure of 10 −5 Torr. The Bi evaporation rate was set to 0.1 nm s −1 , and the Sn evaporation rate was set to 1 nm s −1 , 0.5 nm s −1 and 0.3 nm s −1 to make the Bi x Sn ( x = 0.1, 0.2, and 0.3) samples. The thickness of the deposited Bi x Sn layers was ~700 nm. The pure Bi and Sn films with the same film thicknesses were prepared at an evaporation rate of ~0.3 nm s −1 under the pressure of 10 −5 Torr. Characterization SEM images were taken using a Gemini500 SEM at an accelerating voltage of 2 kV. High-resolution transmission electron microscopy (HRTEM) and transmission electron microscopy-energy dispersive X-ray spectroscopy (TEM-EDX), SAED, and bright-field and dark-field TEM analyses were performed in a TEM (Tecn F20) with an accelerating voltage of 200 kV. X-ray photoelectron spectroscopy (XPS) studies were performed using PHI5000 VersaProbe. The binding energy data were calibrated relative to the C 1s signal at 284.6 eV. In the XPS depth profile studies, the etched depth is ~3–5 nm in each round of the soft Ar etching. X-ray powder diffraction (XRD) was carried out with a Bruker D8 Advance X-ray diffractometer using Cu Kα radiation at a scanning rate of 9°/min in the 2 θ range from 20° to 80°. Electrochemical experiments The CO 2 R experiments were performed in the KHCO 3 and KOH electrolytes in a flow-cell device with a three-electrode setup. Different volumes of 10 M KOH were added to 1 M KHCO 3 solution to adjust the pH to 11, 12, 13, and 14, respectively, confirming with a pH meter. An Ag/AgCl (in saturated KCl) electrode was used as a reference electrode; a nickel foam was used as a counter-electrode; Sn, Bi, and Bi x Sn electrodes were used as working electrodes. The three electrodes were connected to an electrochemical workstation (Metrohm Autolab). The flow rate of CO 2 was set to 20–50 mL min −1 . under standard conditions at the outlet end of the flow cell for all the experiments. The gaseous products were quantified using gas chromatography (GC, PerkinElmer) with a thermal conductivity detector (TCD) and a flame ionization detector (FID). The liquid products were detected using nuclear magnetic resonance (NMR, Bruker 400 M) with water peak suppression. To determine the Faraday efficiency of the liquid products, we quantified the liquid products in both analytes and catholyte by NMR. The electrolytes (on both sides) are also replaced at regular time intervals before the NMR tests. The CO 2 R performance of Bi, Sn, and Bi 0.1 Sn catalysts was also evaluated in MEA electrolysers. A commercial CO 2 R MEA electrolyser (Dioxide Materials) was used to accommodate the electrochemical reactions. The MEA electrolyser was composed of anode and cathode flow field plates with a serpentine-configuration flow field of 5 cm 2 for the continuous supply of anolyte (0.1 M KHCO 3 ) and humidified CO 2 to each respective electrode. We used Bi/PTFE, Sn/PTFE, and Bi 0.1 Sn/PTFE as the cathode, an iridium oxide deposited titanium foam as the anode, and a solid-state cation-exchange membrane (CEM) for HCOO – placed in between the cathode and anode. Before the electrochemical testing, the cathode electrodes (Bi, Sn, or Bi 0.1 Sn on PTFE) were taped to the stainless-steel flow field plate by using a copper frame for homogeneously distributing the electrical current. The anode (IrO x on Ti foam) and cathode were physically separated by CEM (NafionTM 117, Fuel Cell Store) in the solid-state CEM-based MEA experiments and by AEM (Sustainion X37-50 membrane) in the AEM-based MEA experiments. Electrolyser bolts were tightened by applying an equal compression torque. Before experiments, the AEM was activated in 1 M KOH for more than 24 h. Upon completion of the electrolyser assembly, the anolyte (0.1 M KHCO 3 ) flowed through the anode with a constant flow rate of 15 mL min −1 , while the humidified CO 2 was supplied from the gas diffusion electrode (GDL) back with a constant flow rate of 60 standard cubic centimetres per minute (sccm). The full-cell potentials are presented without IR correction. The gas samples were examined using GC (PerkinElmer Clarus 680) to calculate the FE of gas products. The liquid product, formate (when collected from the anodic stream from the AEM-based MEA) or HCOO – (when collected from the cathodic stream from the solid-state CEM-based MEA), was collected from the anodic and cathodic streams simultaneously and analysed by an NMR spectroscopy (Agilent DD2 600 MHz) by using dimethylsulfoxide (DMSO) as the internal standard. The FE towards formate or formic acid at each current density was calculated by adding up both anodic and cathodic FEs. More details are discussed in the supplementary information. Density functional theory (DFT) calculation The facets Bi (003), Sn (200), and Sn (101) are primarily exposed in the Bi, Sn, and Bi 0.1 Sn catalysts (Fig. 1 ); these facets were thus used to build the DFT models (Supplementary Fig. 10 , Supplementary Table 1 ). We incorporated 1–8 Bi into 64 Sn crystals, as more than 8 Bi would de-stabilize the Sn crystal structure (Supplementary Figs. 12 – 15 ). All DFT calculations were performed with the Vienna ab initio simulation package (VASP) [43] . The DFT calculation details are included in the Supplementary Information.